Inbreeding causes early death in a passerine bird Inbreeding typically reduces fitness. Related partners may fail to reproduce and any inbred offspring may die early or fail to reproduce themselves. Here we show that inbreeding causes early death in the zebra finch Taeniopygia guttata , and among inbred individuals of the same inbreeding coefficient ( F ), those that die early are more homozygous (estimated from single nucleotide polymorphisms) than those that survive to adulthood. Therefore, we identify two ways by which inbreeding depression may be underestimated in studies of inbreeding. First, a failure to study early life history could mean that the magnitude of inbreeding depression is routinely underestimated. Second, the observation that the most homozygous individuals of the same pedigree F were the least likely to survive to sexual maturity provides evidence that realized inbreeding, estimated from a high density of markers spread throughout the genome, explains variation in survival above and beyond what pedigree-based measures of inbreeding can explain. Inbreeding is commonly associated with reductions in fitness [1] , [2] , [3] , [4] , [5] , [6] , yet reported effects vary. Several studies of birds, for example, have shown strong inbreeding depression on hatching success of eggs [2] , [3] , but the effects of inbreeding at other stages of development are more equivocal; many studies show no effect or even an advantage of inbreeding on offspring survival [7] , [8] , [9] , [10] , [11] , [12] . Failure to detect an effect on juvenile or adult survival may indicate that inbreeding depression is negligible, but the absence of effects at later stages of development may simply be an artefact of intense inbreeding depression at an earlier stage, such that the most inbred (and least fit) individuals are not included when considering later stages of ontogeny. Accurate measures of inbreeding depression over a species' entire life cycle are therefore required to fully understand the effects of inbreeding in a population. Many studies report strong inbreeding depression on 'fertility' of birds (and other taxa [13] ), but 'infertility' is often used synonymously with 'hatching failure', and the meaning of 'infertility' in this context is ambiguous. Infertility usually refers to the failure of offspring to be produced rather than the failure of eggs to be fertilized, but hatching failure may result from either fertilization failure or embryo death. In birds, embryo mortality that occurs in the first 3–4 days of development is not immediately distinguishable from infertility, and yet, the majority of embryo mortality occurs during these early stages [14] . Distinguishing between these two phenomena is vital for a mechanistic understanding of how inbreeding affects reproductive success, because fertilization success is essentially a trait of one or both parents (who are related but not necessarily inbred themselves), whereas embryo survival is an inherent trait of the inbred individual and may therefore be subject to inbreeding depression. Here we report the effects of relatedness (sib–sib compared with unrelated individuals) on fertilization success, as well as the effects of inbreeding on survival from embryo development through to adulthood, using the zebra finch as a model. Our results demonstrate that the observed effect of inbreeding on survival changes throughout development, with considerable mortality occurring at a very early stage. Our results therefore demonstrate that failure to consider all life history stages may lead to an underestimation of the magnitude of inbreeding depression. Fertilization success and offspring survival Sib–sib and unrelated zebra finch pairs produced very similar proportions of fertile eggs. Most pairs from both groups produced fertile eggs only (16/20 (80%) sib–sib pairs, and 63/77 (82%) unrelated pairs, Fisher's exact test, P =0.242). Of the small number of pairs that produced infertile eggs, the proportion per clutch was not significantly higher for sib–sib pairs than unrelated pairs (mean % fertile per clutch±s.e.m.=88.6±18.5 and 90.6±9.2, respectively; z =0.60, degrees of freedom (d.f. )=12, P =0.549; Fig. 1 ). This indicates that the relatedness of individuals does not affect the compatibility of their gametes for fertilization. However, embryo survival (that is, hatching success of fertile eggs) was significantly lower in sib–sib pairs than unrelated pairs (mean % embryo survival per clutch±s.e.m.=25.2±6.4 and 41.4±3.9, respectively; z =2.97, d.f.=96, P =0.003; estimated number of lethal equivalents ( B ; see Methods for an explanation of how this was estimated)=1.99). 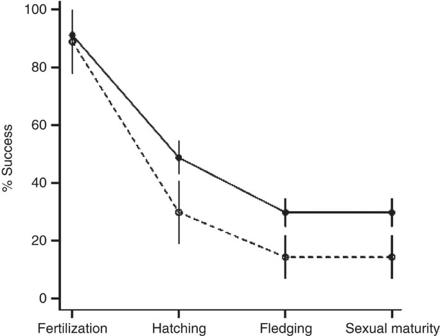Figure 1: Percentage of inbred and non-inbred individuals successfully reaching each life-history stage. Open and closed circles represent inbred and non-inbred individuals, respectively. Error bars show 95% confidence intervals. Data for hatching success are from 1,524 eggs from 329 clutches produced by 97 pairs (of which 20 were sib–sib). Data for fledging success are from 649 chicks that hatched from 228 clutches produced by 82 pairs (of which 14 were sib–sib). Data for survival to sexual maturity are from 333 fledged chicks from 142 clutches produced by 71 pairs (of which 11 were sib–sib). Figure 1: Percentage of inbred and non-inbred individuals successfully reaching each life-history stage. Open and closed circles represent inbred and non-inbred individuals, respectively. Error bars show 95% confidence intervals. Data for hatching success are from 1,524 eggs from 329 clutches produced by 97 pairs (of which 20 were sib–sib). Data for fledging success are from 649 chicks that hatched from 228 clutches produced by 82 pairs (of which 14 were sib–sib). Data for survival to sexual maturity are from 333 fledged chicks from 142 clutches produced by 71 pairs (of which 11 were sib–sib). Full size image More inbred hatchlings died before fledging than non-inbred hatchlings, but this difference (12.4%) was nonsignificant (mean % fledging success per brood±s.e.m.=32.6±10.3 (inbred) and 45.0±4.9 (non-inbred); z =−1.62, d.f.=82, P =0.105; estimated number of lethal equivalents ( B )=1.29). Between fledging and sexual maturity (100 days), there was no mortality in either group; by this stage of development, the earlier difference in survival between the two groups had disappeared ( Fig. 2 ). 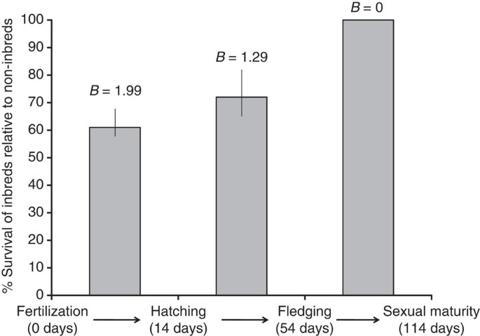Figure 2: Relative survival of inbred compared with non-inbred individuals. Relative survival is presented as % difference between the two cohorts. Error bars show s.e. of the difference. 'Days' are the number of days since fertilization;B=estimated number of lethal equivalents (see Methods). Data for hatching success are from 1,524 eggs from 329 clutches produced by 97 pairs (of which 20 were sib–sib). Data for fledging success are from 649 chicks that hatched from 228 clutches produced by 82 pairs (of which 14 were sib–sib). Data for survival to sexual maturity are from 333 fledged chicks from 142 clutches produced by 71 pairs (of which 11 were sib–sib). Figure 2: Relative survival of inbred compared with non-inbred individuals. Relative survival is presented as % difference between the two cohorts. Error bars show s.e. of the difference. 'Days' are the number of days since fertilization; B =estimated number of lethal equivalents (see Methods). Data for hatching success are from 1,524 eggs from 329 clutches produced by 97 pairs (of which 20 were sib–sib). Data for fledging success are from 649 chicks that hatched from 228 clutches produced by 82 pairs (of which 14 were sib–sib). Data for survival to sexual maturity are from 333 fledged chicks from 142 clutches produced by 71 pairs (of which 11 were sib–sib). Full size image Individual genetic variation and survival Inbred individuals that died between hatching and fledging had significantly higher marker-based F (mean±s.e.m.=0.01±0.06 (died) and −0.02±0.04 (survived); t =2.90, d.f.=10, P =0.027, estimated effect size (d)=0.64) and significantly lower estimated heterozygosity (mean±s.e.m.=0.86±0.05 (died) and 0.96±0.03 (survived); t =3.42, d.f.=10, P =0.016, estimated effect size (d)=0.74) compared with individuals that survived to sexual maturity, despite having the same pedigree F (0.25). Our results suggest that, while individual relatedness does not affect the likelihood of fertilization success, a strong early selection event during embryo development removes the poorest quality inbred individuals, leaving only a relatively 'high-quality' subset of the inbred cohort to hatch. Levels of individual genetic variation estimated from single nucleotide polymorphism (SNP) data were consistent with the hypothesis that 'high-quality' inbred individuals survive longer. The rationale for using SNP data to address this question is as follows. Inbreeding depression mostly arises due to the expression of deleterious recessive alleles, because inbreeding increases the proportion of an individual's genome that is homozygous. Although pedigree-based methods predict F , they fail to account for the fact that among individuals of the same F , there will be variation in homozygosity. This is because although the full-sib parents of our inbred birds had an expected genetic relatedness of 0.5, theoretically they may have shared zero, one or two alleles identical by descent at each locus [15] . The two SNP-based measures of inbreeding distinguish between individuals of the same F that vary in their homozygosity. This indicates that pedigree-based inferences of F , which provide an estimate of the expected genome-wide homozygosity, can be less informative than marker-based approaches, which estimate realized homozygosity. In other words, markers can distinguish between individuals of the same inbreeding coefficient who are more or less homozygous than expected, given their pedigree. In conclusion, we have shown that the effect of inbreeding on zebra finch survival is not consistent across development, due to high mortality at a very early stage. If we are to fully understand the consequences of inbreeding for a population, it is crucial that all developmental stages are considered; otherwise, estimates of inbreeding depression may provide a biased or erroneous picture. This problem may be exacerbated, if inbred individuals that survive early mortality events are less homozygous than expected, given their pedigree-inbreeding coefficient. In particular, studies, where life history stages before hatching (or birth) are ignored, may fail to detect the consequence of inbreeding even when it is present. General The zebra finches used in this study were from a captive population in which baseline levels of inbreeding do not differ significantly from that of wild populations [16] , [17] . Captive birds were used to avoid two main difficulties associated with the study of inbreeding in wild bird populations. First, levels of inbreeding are generally low [18] , [19] , leading to low power. and second, true patterns of male-female reproductive success may be masked by extra-pair paternity [20] . 'Sib–sib' pairs ( n =20) comprised full-sib, non-broodmate individuals; 'unrelated' pairs ( n =77) did not share any grandparents. All eggs were fostered to unrelated parents on the day they were laid. We used the techniques described by Birkhead et al . [21] to distinguish between fertile and infertile eggs. Infertile eggs are those where a sperm pronucleus has not fused with the female pronucleus, and therefore no zygote is formed. Fertilization success of eggs, hatching success of fertile eggs, hatchling survival until fledging (40 days) and survival of fledglings to sexual maturity (100 days) was recorded for all pairs. Estimation of inbreeding load To enable comparisons with other datasets on inbreeding depression, the number of lethal equivalents per gamete ( B ) was estimated. Because data were collected only for non-inbred birds and one class of inbred birds ( F =0.25), a regression of the logarithm of survivorship on inbreeding coefficient is not possible. However, it is still possible to estimate B using equation 10.21b of Lynch & Walsh [5] , where by B =−ln( S f /S o )/ f where S f and S o are the proportions of inbred and outbred birds that survived, and f is the inbreeding coefficient of the inbred birds (here f =0.25). SNP genotyping To assess the effect of homozygosity on fitness, progeny from sib–sib ( n =33) and unrelated matings ( n =42) were genotyped. A panel of 384 SNPs was selected from a larger set of 876 markers that had been successfully typed and mapped in an earlier linkage mapping study [22] . The 384 SNPs were chosen based on Illumina assay design scores, and to get good coverage across the genome, they were located across 35 different chromosomes. Genotyping was performed using custom Veracode GoldenGate kits on an Illumina BeadXpress platform. Genotypes were called using the Illumina Genome Studio Genotyping Module v1.0. A total of 368 SNPs were scoreable, of which 348 were polymorphic. Each bird was scored at a mean (s.d.) of 328 (31) loci. The mean (s.d.) minor allele frequency of each SNP was 0.28 (0.14). Analysis of SNP data We estimated two possible predictors of inbreeding depression from the SNP data: First, we estimated standardized heterozygosity, which is simply the proportion of markers an individual was heterozygous at, scaled by the average heterozygosity of those markers at which it was typed. When the number of markers and the variance in inbreeding coefficient are both relatively large (as is the case here), this measure is a reliable surrogate for inbreeding coefficient [23] . Second, we used a more formal method for estimating inbreeding coefficient from SNP data, using the method based on the diagonals of the adjusted unified additive relationship matrix, described in Powell et al [24] . and implemented within the GCTA software [25] . Statistical analysis All statistical analyses were carried out using R Version 2.10.0 (ref. 26 ). The effects of inbreeding on reproductive success (fertilization, hatching, fledging and survival to sexual maturity) were analysed, using generalized linear mixed models (GLMMs) with inbreeding as a fixed effect, clutch nested within parental pair as random effects, and a binomial error distribution with logit link function (owing to the binary response variable, for example, hatch/not hatch). The majority of eggs were fertile; therefore after comparing the number of pairs that laid any infertile eggs in each group (using Fisher's exact tests), only data from pairs that laid both fertile and infertile eggs were included in the GLMM for fertilization success. Estimates of heterozygosity and marker-based inbreeding coefficients (from SNP data) were also analysed, using GLMMs, with the survival of inbred individuals as a fixed effect and parental pair as a random effect (the 33 inbred individuals included in these analyses were from 10 different families). How to cite this article: Hemmings, N. L. et al . Inbreeding causes early death in a passerine bird. Nat. Commun. 3:863 doi: 10.1038/ncomms1870 (2012).